Epitaxial lift-off process for gallium arsenide substrate reuse and flexible electronics Epitaxial lift-off process enables the separation of III–V device layers from gallium arsenide substrates and has been extensively explored to avoid the high cost of III–V devices by reusing the substrates. Conventional epitaxial lift-off processes require several post-processing steps to restore the substrate to an epi-ready condition. Here we present an epitaxial lift-off scheme that minimizes the amount of post-etching residues and keeps the surface smooth, leading to direct reuse of the gallium arsenide substrate. The successful direct substrate reuse is confirmed by the performance comparison of solar cells grown on the original and the reused substrates. Following the features of our epitaxial lift-off process, a high-throughput technique called surface tension-assisted epitaxial lift-off was developed. In addition to showing full wafer gallium arsenide thin film transfer onto both rigid and flexible substrates, we also demonstrate devices, including light-emitting diode and metal-oxide-semiconductor capacitor, first built on thin active layers and then transferred to secondary substrates. Gallium arsenide (GaAs), with its high electron mobility and direct bandgap, has been employed in high performance RF electronics and optoelectronics for decades [1] , [2] , [3] , [4] . On the basis of thermodynamics calculation, its bandgap lies at the energy for the theoretical maximum efficiency of single junction (SJ) solar cells and makes it an ideal material for high efficiency solar cells [5] . However, the high cost of GaAs substrates hinders them from being widely adopted in certain applications, in particular for solar cell because of a need for large amounts of the material. A typical thickness of a GaAs substrate is around a few hundred micrometres, and only a few micrometres or nanometres thickness is required to fully absorb the solar energy or serve as the active layer for device operation. Therefore, the material cost can be potentially reduced if thin device layers can be separated from the substrate while keeping the substrate intact and ready for another epitaxial growth. In 1978, Konagai et al . [6] proposed a method which is known today as epitaxial lift-off (ELO) to separate a device layer from a GaAs substrate by using hydrofluoric acid (HF) to selectively etch a AlGaAs (aluminium compound) sacrificial layer inserted between the device film and the substrate ( Fig. 1(a) ). Subsequently, this same method has been applied by many researchers to successfully peel GaAs thin films from the parent substrates and transfer them onto desirable substrates for various applications [7] , [8] . The major drawback of this method arises from the high surface roughness of the parent substrate as well as reaction residues left on the substrate after the ELO process, and post-process steps, for example, chemical-mechanical-polish or chemical etching, typically required to reclaim the substrate [9] . In addition, HF is a lethal and highly corrosive acid requiring special handling and extra protection. Compared with typical short processing times with HF in silicon industry, the conventional ELO process takes hours to complete, which potentially increases the exposure risk for operators and the operating cost. Hence, developing a new ELO process with different chemistry that enables the direct reuse of the substrate is very desirable to lower the overall cost. Although HCl-based etchant was proposed and used by several researchers to selectively etch AlGaAs [10] , [11] or other sacrificial layers [12] , [13] , [14] , the possibility of reusing the substrate directly with these methods has not been explored. In this paper, we demonstrate a new ELO process where aluminium-arsenide based sacrificial layer and HF-based etchant are replaced with phosphide-based materials and HCl. This new approach minimizes the amount of post-etching residues and provides the surface passivation that keeps the surface smooth during ELO process, leading to direct reuse of GaAs substrate. 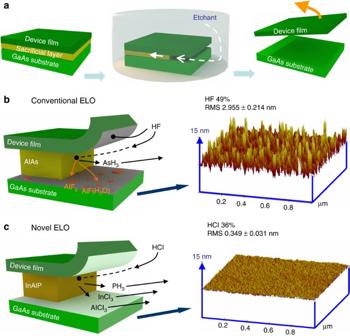Figure 1: Concept of epitaxial lift-off (ELO) process and post-ELO GaAs surface morphologies with conventional and novel ELO processes. (a) Schematic illustration of general ELO process. (b,c) Schematic illustrations of the chemical reactions near the sacrificial layer/etchant interfaces during the conventional and the novel ELO process and the three-dimensional AFM images of the GaAs surfaces after the processes. Here, indium aluminium phosphide (InAlP) was taken as an example of the sacrificial layer of the novel ELO process. Figure 1: Concept of epitaxial lift-off (ELO) process and post-ELO GaAs surface morphologies with conventional and novel ELO processes. ( a ) Schematic illustration of general ELO process. ( b , c ) Schematic illustrations of the chemical reactions near the sacrificial layer/etchant interfaces during the conventional and the novel ELO process and the three-dimensional AFM images of the GaAs surfaces after the processes. Here, indium aluminium phosphide (InAlP) was taken as an example of the sacrificial layer of the novel ELO process. Full size image Mechanism of the ELO Process for reuse of GaAs substrates A viable ELO process for manufacturing should satisfy three essential conditions: (1) the surface of the reused substrate needs to be residue-free, and have low surface roughness (the root-mean-square (RMS) roughness of an epi-ready GaAs wafer is about 0.3 nm); (2) the properties of subsequent layers grown on reused substrates should be identical to that of the first released film; (3) the throughput of the ELO process should be high to drive down overall cost. Fig. 1(b) illustrates the chemical reactions of the conventional ELO process and atomic-force microscopy (AFM) image of the post-ELO substrate surface. The attack of the substrate by the HF and the residues formed during the sacrificial layer etching result in the increase of RMS roughness from 0.3 to 1–4 nms range. Chemical reactions between AlAs and HF have been well studied [10] , [15] , [16] and the two major reactions are shown below: Three primary byproducts from these etching reactions are AlF 3 , [AlF n (H 2 O) 6− n ] (3− n )+ and AsH 3 . AsH 3 is gaseous and can form bubbles and diffuse away from the interface to the atmosphere. AlF 3 and [AlF n (H 2 O) 6− n ] (3− n )+ , on the other hand, are solid and hard to dissolve into the solution. Besides these primary byproducts, solid As 2 O 3 can also be generated on the substrate depending on the oxygen concentration of the etchant [17] . Table 1 summarizes the solubility of the solid byproducts from the conventional ELO process [18] . Although AlF 3 and As 2 O 3 do not have extremely low aqueous solubilities, it is evident that they still remain on the substrate surface after ELO and cause a high surface roughness, which can be seen in Fig. 1(b) . Moreover, HF used in this process slowly attacks GaAs and induces additional surface roughness. Post-chemical etching with thermal cleaning can potentially reduce the surface roughness to the level of the original wafer. However, the remaining contaminants still seriously degrade the quality of regrown films and device performances [9] . To completely remove all these contaminants and achieve high quality regrown films, multi-step chemical polishing with different sacrificial (protection) layers was recently proposed, with the penalties of the higher cost for extra epitaxial growths and HF still being used as the main etchant [19] . Table 1 Solubility of etching products from conventional and novel ELO process. Full size table The abovementioned issues in the conventional ELO process can be mitigated by employing a different sacrificial layer that can be selectively etched by a non-HF solution, while leaving no insoluble etching byproducts on the GaAs surface. One advantage of compound semiconductors is that their physical and chemical properties can be manipulated by alloying different group III and V elements. For example, phosphide-based materials (InGaP, InAlP, InP and so on) have been widely applied as etch stop layers for the selective etching of arsenide based materials (GaAs, InGaAs and so on), and vice versa. It is well known that hydrochloric acid (HCl) can etch phosphide-based materials [14] , [20] , [21] , [22] and the reaction is shown in Equation (3): The gaseous PH 3 diffuses away from the interface and the rest of the etching byproducts are highly soluble (their solubilities are shown in Table 1 ); thus, no residues are left on the wafer surface. Fig. 1(c) illustrates the new ELO process and AFM image of the post-ELO surface. The wafer surface is atomically flat with RMS roughness of merely 0.349 nm—significantly improved over conventional ELO ( Supplementary Fig. S1 ). This improvement comes from the almost infinite etch-selectivity between GaAs and phosphide with the HCl etchant. In order to verify that HCl attacks GaAs much less compared with HF, we soaked blanket GaAs wafers in HCl or HF for 24 h and the AFM images afterwards are shown in Fig. 2(a) . RMS roughness of the 24h-HCl wafer is only 0.327 nm, much lower than the 1.666 nm RMS roughness after 24 h in HF. This result indicates that HF attacks GaAs severely and causes excess surface roughness even without the ELO process. This can be explained through possible etching mechanisms for GaAs with HF and HCl, as shown in Equation (4). In contrast to the etching of GaAs by HF that is thermodynamically favourable (ΔG <0), the reaction with HCl is suppressed (ΔG >0) [18] . 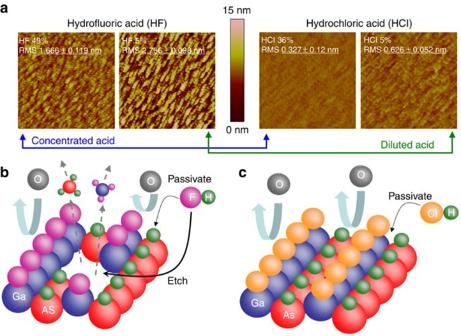Figure 2: Surface morphologies of GaAs surfaces during ELO process. (a) AFM images of the GaAs substrate surface dipped in both concentrated and diluted HF and HCl for 1 day. (b,c) are the schematic illustrations of the surface chemistry of GaAs dipped in HF and HCl, respectively. Figure 2: Surface morphologies of GaAs surfaces during ELO process. ( a ) AFM images of the GaAs substrate surface dipped in both concentrated and diluted HF and HCl for 1 day. ( b,c ) are the schematic illustrations of the surface chemistry of GaAs dipped in HF and HCl, respectively. Full size image Therefore, the etch rate of GaAs in HCl is much lower and the surface remains smoother. Note that in the particular alloy example in Equation (3), aluminium is not required for selective etching, but it can accelerate etching of the sacrificial layer. Moreover, because only undissociated HCl molecules interact with phosphide, the throughput is greatly enhanced by using concentrated HCl with the new ELO process [20] , [23] , [24] . The use of HCl as an etchant also poses significantly lower risks compared with highly lethal and corrosive HF. These attributes makes the new ELO process much safer and economical for manufacturing compared with the conventional method. In addition to reducing substrate etching to minimize surface roughness, surface passivation of GaAs by acids also has an important role. Fig. 2(a) shows that GaAs wafers soaked in diluted acids display higher RMS roughness than those soaked in concentrated acids. It is well known that the combination of acid or base with oxidants can be an effective GaAs etchant and dissolved oxygen can serve as an oxidant. On the other hand, both HF and HCl can passivate the surface and prevent it from being oxidized by dissolved oxygen ( Supplementary Fig. S2 and Supplementary Methods ). The competition between surface passivation by acids and etching by dissolved oxygen determines the surface roughness at different acid concentrations. These processes are illustrated in Fig. 2(b . It has been proven that the GaAs surface becomes highly hydrophobic (like H-terminated surface that forms by dipping Si into HF) after it is dipped into HF or HCl [25] , [26] . The surface gallium atoms are passivated by fluorine or chlorine atoms and the surface arsenic atoms are possibly passivated by hydrogen atoms [25] , [27] , [28] , [29] . Higher acid concentrations provide better coverage of passivated atoms and leave fewer unprotected sites to be oxidized by dissolved oxygen. The main difference between HCl and HF is that HCl only passivates the surface while HF not only passivates the surface, but slowly etches the bulk GaAs. In order to verify the hypotheses discussed above, a GaAs sample was placed into diluted (5%) HCl purged with pure N 2 to release dissolved oxygen from the solution for 2 days( Supplementary Fig. S3 and Supplementary Methods ). The final surface roughness is 0.358 nm and is almost identical to the GaAs sample soaked in concentrated HCl for 1 day, suggesting that dissolved oxygen in diluted HCl roughens the surface. To quantify the etch rates of GaAs with HCl and HF, GaAs samples were left in 36% HCl, 5% HF and 49% HF for 9 days. The etch depths were measured to be 3, 12 and 100 nm, respectively, ( Supplementary Fig. S4 and Supplementary Methods ). We attribute the minor etching of 36% HCl to dissolved oxygen in HCl and confirm the significantly higher GaAs etch rate in HF. Demonstration of substrate reuse As a smooth surface does not guarantee re-usability of the wafer after ELO [9] , SJ solar cell structures were grown and fabricated on both the original substrate and the reused substrate to confirm the quality of the regrown layers. 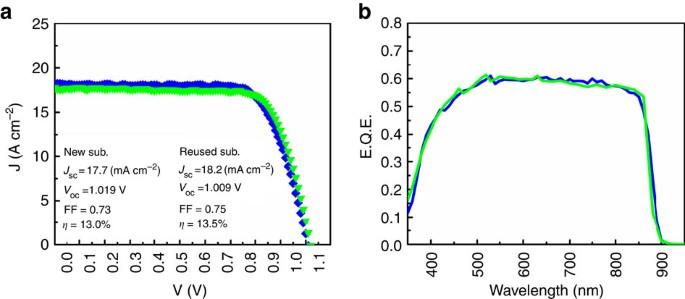Figure 3: Performance of single junction GaAs solar cells fabricated on new and reused substrates. (a) Current density versus voltage (J–V) characteristics of GaAs SJ solar cells grown and fabricated on new (green symbols) and reused (blue symbols) substrates. Inset: solar cell performance parameters. (b) EQE of solar cells grown on new (green) and reused (blue) substrates as a function of wavelength. No anti-reflection coating (ARC) was applied. Figure 3(a) shows current density versus voltage (J–V) characteristics measured under AM1.5 sun condition, and Fig. 3(b) shows the external quantum efficiencies (EQE) of both cells. No substantial difference in short circuit current ( J sc ), open circuit voltage ( V oc ), fill factor (FF), efficiency ( η ) and EQE was observed. We attribute some slight mismatches of solar cell performance to fabrication process variations. The fact that no performance degradation is observed on the cell fabricated on the reused substrate demonstrates the feasibility of direct reuse of GaAs substrates by applying phosphide base sacrificial layer and the use of concentrated HCl as the etchant. Figure 3: Performance of single junction GaAs solar cells fabricated on new and reused substrates. ( a ) Current density versus voltage (J–V) characteristics of GaAs SJ solar cells grown and fabricated on new (green symbols) and reused (blue symbols) substrates. Inset: solar cell performance parameters. ( b ) EQE of solar cells grown on new (green) and reused (blue) substrates as a function of wavelength. No anti-reflection coating (ARC) was applied. Full size image Surface tension-assisted ELO process as a new lift-off method Finally, one major throughput bottleneck in conventional ELO processes is the slow lateral etch rate of the sacrificial layer. Generally speaking, the lateral etch rate of the sacrificial layer is determined by two consecutive processes: the diffusion of the etchant from the solution to the etching front and the reaction of etchant with the sacrificial layer. The etch rate is initially limited by the chemical reaction until the diffusion distance of the etchant causes the etch rate to be limited by the diffusion rate. Performing the ELO process in the chemical reaction rate limited regime is preferred as it can maximize the overall etch rate. In order to do so, several methods with sophisticated setups, for example, weight-assisted ELO [30] and etching assisted by roller [15] , [31] , were developed to accelerate the ELO process. However, these are only single-wafer solutions with consequent low throughput. To enhance our ELO process throughput, we developed a new method called ‘surface tension-assisted (STA) ELO’ and its concept is shown in Fig. 4(a) . The wafer coated with the photoresist is placed obliquely with an angle (θ) of 1°–20° from the solution surface, and HCl is added to the level of the etching front. The wafer surface is protected by the photoresist from being attacked by the acid. As discussed above, the GaAs surface becomes hydrophobic in HCl, so the film floats on the surface of the HCl solution after lift-off. During the STA-ELO process, surface tension pulls the film away from the substrate and flattens the film on the surface. In the meantime, HCl replenishes the space between the lifted-off film and the substrate via the capillary force, which causes the process to continue to be reaction limited. 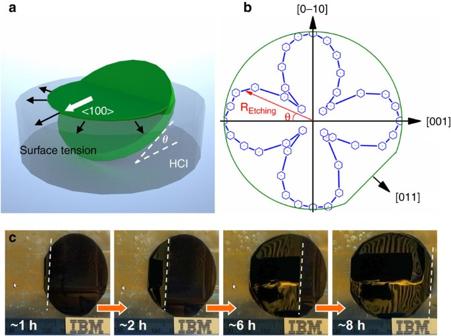Figure 4: Surface tension-assisted ELO process. (a) Schematic illustration of the surface tension-assisted (STA) ELO process. (b) Etching rate of InAlP in HCl as the function of crystallographic direction. The maximum etching rate locates at <100>. All the data were normalized by maximum etching rate. (c) Recorded images of the lifted-off film during STA-ELO process. The minor image distortion was caused by the vibration of hood. The InAlP sacrificial layer thickness is 100 nm.The temperature of HCl solution was kept at 60 °C and the process took about 8 h. The average lateral etching rate is ~5.9 mm h−1in this demonstration. The etching rate could be increased by further optimization of the process, structure and setup. Figure 4(b) shows the relationship between the normalized etch rate of the phosphide sacrificial layer and the crystallographic direction of the wafers. The study reveals a fourfold symmetry where the maximum etch rate occurs along the <100> axis, as the etching fronts are terminated by {111} A faces [32] . As a result, the wafer needs to be tilted along the <100> axis for the highest etch rate and to keep the etching front along the <100> direction. This allows the surface tension of the solution to apply a uniform force on the lifted-off film. The complete STA-ELO process is shown in Fig. 4(c) and in the Supplementary Video S1 . The camera reflection on the lifted-off film demonstrates how the surface tension of the solution results in a flat surface. The lifted-off film can be transferred onto almost any substrate for various applications, including either a rigid ( Fig. 5(a) ) or a flexible substrate ( Fig. 5(b) ). After the ELO process, the parent wafer only needs to be rinsed thoroughly and then cleaned with a standard wafer cleaning procedure before the next epitaxial growth. Figure 4: Surface tension-assisted ELO process. ( a ) Schematic illustration of the surface tension-assisted (STA) ELO process. ( b ) Etching rate of InAlP in HCl as the function of crystallographic direction. The maximum etching rate locates at <100>. All the data were normalized by maximum etching rate. ( c ) Recorded images of the lifted-off film during STA-ELO process. The minor image distortion was caused by the vibration of hood. The InAlP sacrificial layer thickness is 100 nm.The temperature of HCl solution was kept at 60 °C and the process took about 8 h. The average lateral etching rate is ~5.9 mm h −1 in this demonstration. The etching rate could be increased by further optimization of the process, structure and setup. 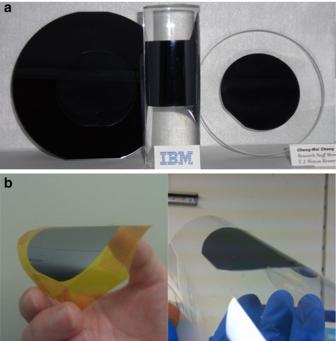Figure 5: GaAs thin films transferred to rigid and flexible substrates. (a) Demonstrations of the transferred GaAs thin films to the rigid Substrate (left, GaAs on 4″ Si wafer. Center, GaAs on curved solid object. Right, GaAs on glass) and (b) flexible substrates (left, GaAs on tape. Right, GaAs on flexible sheet). The thickness of the GaAs ranges between 1–3 μm and the diameter of the GaAs is 2″ except the film transferred to the curved solid object. Full size image Figure 5: GaAs thin films transferred to rigid and flexible substrates. ( a ) Demonstrations of the transferred GaAs thin films to the rigid Substrate (left, GaAs on 4″ Si wafer. Center, GaAs on curved solid object. Right, GaAs on glass) and ( b ) flexible substrates (left, GaAs on tape. Right, GaAs on flexible sheet). The thickness of the GaAs ranges between 1–3 μm and the diameter of the GaAs is 2″ except the film transferred to the curved solid object. Full size image After the STA-ELO process, the GaAs thin film can be transferred onto any thermal-expansion-coefficient (TCE) matched substrates (for example, soda-lime glass) without using any metal supporting layer during ELO process. This helps keep the GaAs surface pristine and the newly transferred film compatible with epitaxy systems for subsequent epitaxial growth. Another advantage is that devices can be fabricated on the GaAs surface first before the film containing the devices is released from the parent substrate. By these means, the device yield can be largely improved, as it reduces the constraint on the highest process temperature allowable imposed by the thermal mismatch between the film and the carrier substrate. 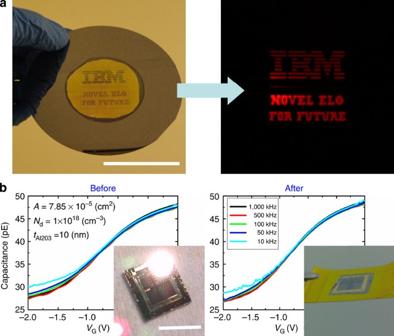Figure 6: Demonstration of transferred devices via novel ELO process. (a) Transferred 2″ AlGaAs LED on 2″ Si wafer and the optical image of light emission. Scale bar, 5 cm. (b) Capacitance–Voltage (C–V) characteristics of n-GaAs MOSCAP before and after being transferred to a flexible tape. Inset: the optical image of MOSCAPs on a mother substrate and on a flexible tape. Scale bar, 1 cm. Figure 6 demonstrates some conceptual devices fully fabricated in advance before our STA-ELO process: (a) a light-emitting diode (LED) transferred onto Si substrate ( Supplementary Fig. S5 ), and (b) metal-oxide-semiconductor capacitors (MOSCAP) transferred onto flexible tape. Red light emission in Fig. 6(a) suggests that the integrity of the LED was preserved after the film transfer. Figure 6(b) shows capacitance–voltage measurements from GaAs MOSCAPs at different frequencies, demonstrating no observable difference between devices measured before and after the thin film transfer. Figure 6: Demonstration of transferred devices via novel ELO process. ( a ) Transferred 2″ AlGaAs LED on 2″ Si wafer and the optical image of light emission. Scale bar, 5 cm. ( b ) Capacitance–Voltage (C–V) characteristics of n-GaAs MOSCAP before and after being transferred to a flexible tape. Inset: the optical image of MOSCAPs on a mother substrate and on a flexible tape. Scale bar, 1 cm. Full size image In conclusion, the direct reuse of GaAs substrates has been demonstrated by a newly developed ELO process. Residue-free and atomically flat post-ELO surfaces, resulting from the use of phosphide base sacrificial layers and HCl-based etchants, results in high quality regrown GaAs thin films and enables the regrowth of solar cell structures without observable performance degradation. Furthermore, STA-ELO, a high-throughput lift-off technique, is developed and employed to transfer GaAs thin films onto both rigid and flexible substrates. This technique opens up a suite of potential applications using III–V materials. Material growth III–V growth, including both arsenide and phosphide base materials, was performed in Thomas Swan close coupled showerhead cold-wall MOCVD system. High-purity N 2 was employed as the carrier gas, and the substrate temperature and the reactor pressure were kept at 650 °C and 100 Torr during the growth. Epilayers were grown on either 2″ n-type (Si doped) or p-type (Zn doped) epi-ready GaAs wafers depending on the device structures. Trimethylgallium (TMG), Trimethylaluminum (TMA) and Trimethylindium (TMI) were used as element III precursors. Arsine (AsH 3 ) and Phosphine (PH 3 ) were used as element V sources for growing arsenide (V/III=23) and phosphide (V/III=400) materials, respectively. DiSilane (Si 2 H 6 ) provided n-type dopants and dimethylzinc was used for p-type doping. Experiment, device fabrication and characterization The layers of III–V solar cells were grown on a 2″ N-type GaAs wafers. The wafers were then cut into two pieces with one piece serving as a reference. The other piece went through ELO process to separate the solar cell structure from the substrate, and it was then reloaded into MOCVD system and the same layer structure was regrown. After the regrowth, these two pieces were processed in parallel to complete the final solar cell structures, which is shown in Supplementary Fig. S6 . A detailed process flow is described below. 1 × 1 cm 2 mesa was defined by photolithography and etched to the bottom contact layer by NH 4 OH/H 2 O 2 /H 2 O. The bottom n-ohmic contact was made with thermal evaporated AuGe/Ni/Au and a lift-off process, followed by rapid-thermal annealing (RTA) at 450 °C for 1 min in N 2 ambient. Then, a shadow mask was applied to define the top p-ohmic contact region by depositing Au/Ni and 1 μm thick Ag to lower the series resistance. After removing the shadow mask, the top contact layer (p-GaAs) was selectively etched by citric acid/H 2 O 2 . No RTA was performed for p-type ohmic contact and no anti-reflection coating was applied on the solar cells. The J–V characteristics of GaAs SJ solar cells were measured under simulated AM1.5 solar spectrum at 1 sun intensity. A similar process flow for the solar cell was applied for LED device fabrication, and the layer structure as well as the final device structure of LED are shown in Supplementary Fig. S7 . MOSCAPs were fabricated by the following process flow. After surface degreasing and ammonia-base native oxide etching, the sample was transferred to an ALD reactor and 10 nm thick Al 2 O 3 was deposited at a substrate temperature of 250 °C, followed by 600 °C post-deposition annealing for 15s. The substrate contact was defined by photolithography and Al 2 O 3 was removed by buffered oxide etch (BOE) solution and n-ohmic contact was made by thermal evaporated AuGe/Ni/Au and a lift-off process, followed by N 2 RTA at 450 °C for 1 min. Top Al electrodes of 100 μm in diameter were deposited by thermal evaporation through a shadow mask. Finally, the fabricated MOSCAPs were transferred onto a piece of flexible tape. C–V characteristics of MOSCAP were measured using Agilent 4284A precision LCR metre at frequencies from 1 MHz to 10 kHz. The layer structure and the final MOSCAP structure are shown in Supplementary Fig. S8 . How to cite this article: Cheng, C.-W. et al . Epitaxial lift-off process for gallium arsenide substrate reuse and flexible electronics. Nat. Commun. 4:1577 doi: 10.1038/ncomms2583 (2013).